SMRT compounds abrogate cellular phenotypes of ataxia telangiectasia in neural derivatives of patient-specific hiPSCs Ataxia telangiectasia is a devastating neurodegenerative disease caused primarily by loss of function mutations in ATM , a hierarchical DNA repair gene and tumour suppressor. So far, murine models of ataxia telangiectasia have failed to accurately recapitulate many aspects of the disease, most notably, the progressive cerebellar ataxia. Here we present a model of human ataxia telangiectasia using induced pluripotent stem cells, and show that small molecule read-through compounds, designed to induce read-through of mRNA around premature termination codons, restore ATM activity and improve the response to DNA damage. This platform allows for efficient screening of novel compounds, identification of target and off-target effects, and preclinical testing on relevant cell types for the pathogenic dissection and treatment of ataxia telangiectasia. A-T (ataxia telangiectasia) is an autosomal recessive genetic disease caused by mutations in the ATM gene [1] , [2] , [3] , [4] . Clinically, A-T patients are characterized by progressive childhood cerebellar ataxia, the most notable phenotype, as well as radiosensitivity, immunodeficiency and cancer susceptibility [5] . The ATM gene encodes a serine/threonine kinase with a hierarchical role in the double-strand break (DSB)-triggered DNA damage response [6] . Pathological mutations in ATM lead to the loss of protein and/or its kinase activity, which contributes to the pleiotropic phenotypes of A-T [7] . More than 700 mutations have been identified for A-T patients, including nonsense, splicing, frameshift and missense [8] . Currently, no long-term disease-altering treatment is available for A-T patients [9] . Mutation-targeted therapies, such as read-through compounds (RTCs) for nonsense mutations [10] , [11] , [12] and antisense morpholino oligonucleotides for splicing mutations [13] , [14] , [15] , have restored functional expression of the ATM protein in A-T patient-derived cells. Several leading RTCs from our previous studies induced expression of functional ATM protein in human nonsense mutation-containing lymphoblastoid cell lines (LCLs) and fibroblasts derived from A-T patients [11] . However, the tested cells were not the most relevant cell targets for A-T treatment, as cerebellar neural cells are thought to be the primary targets for abrogating neurodegeneration in patients. Furthermore, Atm knockout (Atm−/−) mice do not manifest the progressive ataxia seen in A-T patients and also fail to show marked loss of Purkinje cells (PCs) in the cerebellum, currently believed to be a hallmark of the ATM -related neural deficits observed in disease [16] , [17] , [18] . Thus, development of a human neural cell model is crucial for the study of cerebellar neurodegeneration in A-T patients as well as for testing new therapeutic approaches. Human induced pluripotent stem cells (hiPSCs) represent a promising paradigm with which to model neural differentiation and degeneration, and perhaps even the role of ATM as a tumour suppressor in cell culture. In theory, hiPSCs have the capacity to differentiate into the entire spectrum of neurons, including PCs. Therefore hiPSC-derived neural cells could serve as ideal models for drug development, pharmacokinetic analyses, and targeting inherited neural disorders. In this study, we demonstrate that hiPSC-derived neural cells from A-T patients display hallmarks of the disease in vitro and the physiological defects can be abrogated through the use of small molecule read-through (SMRT) compounds. Generation of A-T patient-specific neural derivatives To develop a cell based, in vitro model of clinically relevant cell types for A-T, fibroblasts from patients with either a nonsense (A-T-Nons) or splicing (A-T-Spl) mutation were reprogrammed to the pluripotent state. Briefly, a polycistronic virus bearing human versions of the Yamanaka factors ( OCT4, SOX2, KLF4 and CMYC ) was used to infect WT, nonsense (homo:103C>T) or splicing (Het: (a)967A>G;(b)3802delG) fibroblasts. A week later, the infected cells were transferred to hESC growth conditions [19] . After colony formation and verification by Tra1-81 staining, clones were expanded and lines derived from each experiment. This led to the generation of several distinct hiPSC lines per fibroblast line reprogrammed. The results of the reprogramming are displayed in Fig. 1 . The reprogrammed lines expressed high levels of human pluripotent stem cell markers OCT4, SOX2, TRA1-81 and NANOG ( Fig. 1a ). Furthermore, after injection of 5 × 10 6 cells of each line into immunocompromised mice (NOD-SCID), each was able to form teratomas, demonstrating the pluripotency of the WT and A-T hiPSC lines ( Fig. 1b ). Finally, DNA sequencing indicated that the hiPSC lines generated carried the expected mutations originally found in the fibroblasts that were reprogrammed (data not shown). 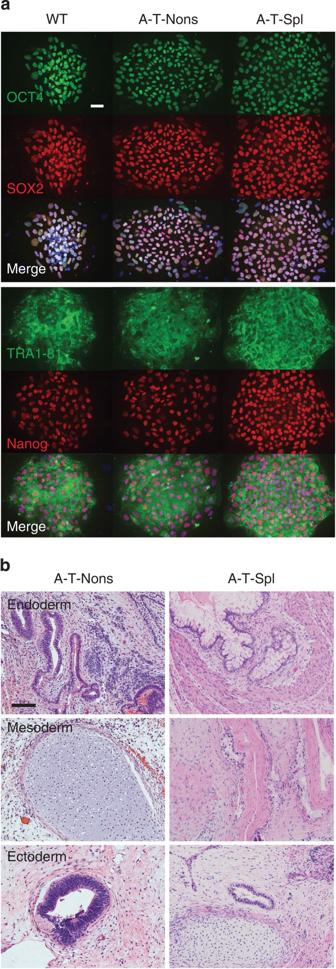Figure 1: Generation of hiPSC lines from A-T fibroblasts. (a) After addition of a polycistronic reprogramming vector bearing the Yamanaka factors, infected fibroblasts were seeded onto feeder plates under hESC growth conditions. Colonies formed 4–9 weeks later. Promising colonies were picked, replated and cell lines generated such as those shown. Each of these cell lines stained positively for OCT4, SOX2, Tra1-81 and NANOG. Scale bar, 50 μm. (b) To demonstrate that the reprogrammed cell lines were pluripotent, 5 million cells of each line were injected into various portions of immunocompromised mice. In every case, the lines described in this paper formed teratoma tumours, which each displayed evidence of derivatives from all three embryonic germ layers (ectoderm, endoderm, mesoderm) indicating their pluripotency. Scale bar, 50 μm. Figure 1: Generation of hiPSC lines from A-T fibroblasts. ( a ) After addition of a polycistronic reprogramming vector bearing the Yamanaka factors, infected fibroblasts were seeded onto feeder plates under hESC growth conditions. Colonies formed 4–9 weeks later. Promising colonies were picked, replated and cell lines generated such as those shown. Each of these cell lines stained positively for OCT4, SOX2, Tra1-81 and NANOG. Scale bar, 50 μm. ( b ) To demonstrate that the reprogrammed cell lines were pluripotent, 5 million cells of each line were injected into various portions of immunocompromised mice. In every case, the lines described in this paper formed teratoma tumours, which each displayed evidence of derivatives from all three embryonic germ layers (ectoderm, endoderm, mesoderm) indicating their pluripotency. Scale bar, 50 μm. Full size image Previous work showed decreased reprogramming efficiency and genomic instability in tm-null murine cells [20] . Here, we also found that reprogramming two different human ATM-mutant somatic cell lines did occur at a somewhat reduced efficiency and took longer on average than wild-type cells (4–5 weeks in WT; 6–9 weeks in AT-mutant), further suggesting that active DNA repair machinery is important for reprogramming. In addition, we did detect aneuploidy in some AT-patient derived FBs or in neural progenitor cells (NPCs) derived therein ( Supplementary Figs S1 and S2 ). Both traditional karyotyping and a newer method that allows for karyotypic abnormalities to be predicted from RNA expression data mapped to the genome [21] , [22] were applied ( Supplementary Figs S1 and S2 ). Traditional karyotyping on the AT-FBs used for reprogramming showed abnormalities in a fraction of the starting pool of (GM01588) cells, while the resulting NPCs produced after reprogramming did not show any abnormalities ( Supplementary Fig. S1 ). This suggests that reprogramming only occurred in the fraction of starting cells with a normal karyotype, which could perhaps explain the low efficiency of reprogramming for that patient derived line. In AG04405 cells, the FBs appeared to be karyotypically normal, but a fraction of the NPCs produced from the corresponding hiPSCs contained an inversion event on Chromosome 3 ( Supplementary Fig. S1 ). Karyotpying based on gene expression analysis did not find any aneuploidy events, as this method is limited to detection of aneuploidy that exists only when at least 30% of cells in the pool have the aberration ( Supplementary Fig. S2 ). Both of these analyses suggested that loss of ATM does correspond with genomic instability, as has been described previously [20] . In addition, neither of these analyses excluded the possibility that smaller, subkaryotpyic abnormalities may exist in any of these lines. Future work will employ array competitive genomic hybridization (CGH) and direct sequencing to identify whether loss of ATM leads to significant genomic abnormalities even in the absence of irradiation-induced DNA damage. As A-T is a disease that affilcts the central nervous system, specifically Purkinje neurons of the cerebellum, established methods were employed to drive the WT and A-T hiPSCs towards neural lineages. NPCs were generated and expressed all the typical hallmarks such as SOX2 and NESTIN ( Fig. 2a ). To ensure the authenticity of NPCs generated from WT and A-T hiPSCs lines, gene expression profiling of hiPSCs, NPCs and fibroblasts was performed. Indeed, NPCs derived from A-T patient fibroblasts clustered with NPCs derived from WT hiPSC and hESC lines, and were distinct from other cell types ( Fig. 2b ). Furthermore, NPC marker genes were highly specific to the NPCs produced at both protein ( Supplementary Fig. S2A ) and RNA ( Supplementary Fig. S2B ) level, confirming their identity as bona fide NPCs. Immunostaining and western blotting for total ATM protein showed that NPCs made from two distinct mutant A-T fibroblast lines failed to express ATM protein as expected ( Fig. 2c ). 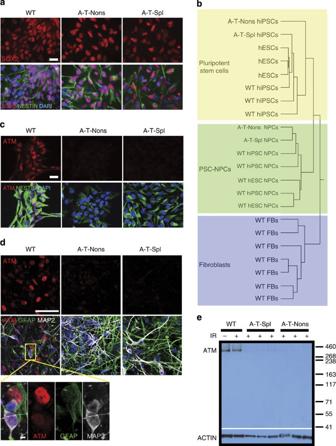Figure 2: hiPSC lines from A-T patients generated neural derivatives that lack expression of ATM protein. (a) NPCs from WT, A-T-Nons and A-T-Spl were stained for typical markers SOX2 and NESTIN. Scale bar, 20 μm. (b) To broadly characterize the nature of NPCs made from A-T patients, the NPCs were transcriptionally profiled by microarray and compared with numerous WT-NPCs. Hierarchical clustering based on transcriptional similarity indicated that these werebona fideNPCs, clearly distinguished from pluripotent stem cells or fibroblasts. (c) A-T-NPCs lacked ATM protein expression as measure by immunostaining. Scale bar, 20 μm. (d) WT and A-T-NPCs were further differentiated to neurons (MAP2) and astrocytes (GFAP) by the withdrawal of growth factors. In this case, both astrocytes and neurons from A-T patients lacked ATM protein expression by immunostaining. Scale bar, 50 μm in main panel, Scale bar, 10 μm for the inset. (e) Western blotting of A-T-NPC whole-cell lysates indicated a lack of ATM protein, and that the antibody used incanddwas highly specific for ATM. Figure 2: hiPSC lines from A-T patients generated neural derivatives that lack expression of ATM protein. ( a ) NPCs from WT, A-T-Nons and A-T-Spl were stained for typical markers SOX2 and NESTIN. Scale bar, 20 μm. ( b ) To broadly characterize the nature of NPCs made from A-T patients, the NPCs were transcriptionally profiled by microarray and compared with numerous WT-NPCs. Hierarchical clustering based on transcriptional similarity indicated that these were bona fide NPCs, clearly distinguished from pluripotent stem cells or fibroblasts. ( c ) A-T-NPCs lacked ATM protein expression as measure by immunostaining. Scale bar, 20 μm. ( d ) WT and A-T-NPCs were further differentiated to neurons (MAP2) and astrocytes (GFAP) by the withdrawal of growth factors. In this case, both astrocytes and neurons from A-T patients lacked ATM protein expression by immunostaining. Scale bar, 50 μm in main panel, Scale bar, 10 μm for the inset. ( e ) Western blotting of A-T-NPC whole-cell lysates indicated a lack of ATM protein, and that the antibody used in c and d was highly specific for ATM. Full size image The array data were also used to determine whether the absence of ATM protein or any resulting genomic instability caused any broad transcriptional differences in hiPSCs or NPCs ( Fig. 2 ). A number of genes did show up as statistically different between WT and AT-patient derived cells ( Supplementary Data 1 ). However, gene onotology analysis identified just a handful of unique functional categories, and only in hiPSCs lacking ATM ( Supplementary Table S1 ), while no categories were defined in NPCs ( Supplementary Fig. S3C ). Next, the NPCs from WT and A-T hiPSC lines were then further differentiated to neurons and glia by growth factor withdrawal [23] , [24] ( Fig. 2d ). All hiPSC lines analysed were capable of producing both neurons (MAP2+) and glia (GFAP+) within 3 weeks, and A-T lines showed a lack of ATM protein expression in these differentiated post-mitotic neural cell types ( Fig. 2d ). Altogether, these findings suggest that ATM protein does not have a significant role in neural differentiation in this setting. A human cell-based molecular phenotype for A-T ATM is activated rapidly by auto-phosphorylation in response to DNA damage [25] . Thus, activation of ATM kinase activity was measured after gamma irradiation (IR) to establish a basic A-T cellular phenotype in patient-derived NPCs. WT-NPCs showed a clear induction of ATM-pS1981 nuclear foci 30 min after IR (2 Gy) as expected ( Fig. 3a ). In contrast, A-T-NPCs failed to show any post-IR activation of ATM kinase ( Fig. 3a ). A similar IR-induced activation of ATM was observed in WT-NPC lines when ATM-pS1981 activation was measured by FACS ( Fig. 3b ). ATM activity was also assessed by measuring phosphorylation of downstream targets, such as SMC1 ( [26] , [27] ). SMC1 activity can be measured with an antibody to the phosphorylated version of the protein (SMC1pSer966) and subsequent FACS analysis. WT-NPCs showed strong activation of SMC1pS966 30 min after gamma irradiation, while both A-T-NPCs lines showed negligible activation similar to our previous studies with LCLs [28] , [29] ( Fig. 3c ). 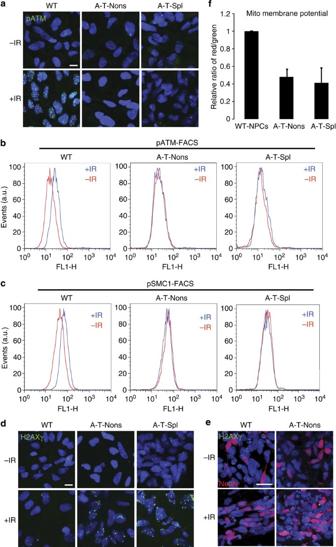Figure 3: Neural derivatives of A-T hiPSCs display physiological deficits common to A-T cellular phenotype. (a) In WT-NPCs, induction of DNA damage by IR (2 Gy) led to phosphorylation of ATM at 30 min, as indicated by immunostaining. Conversely, A-T-NPCs lacked substantial ATM phosphorylation at this time point. Scale bar, 2 μm. (b) The phosphorylation of ATM was also measured by FACS. Again, A-T-NPCs failed to induce pATM with this assay as judged by the mean fluorescence intensity across all cells in the culture29. (c) SMC1, a direct target of ATM phosphorylation, was measured by FACS and presented as mean fluorescence intensity across all cells. A-T-NPCs did not show appreciable levels of SMC1 phosphorylation. (d,e) Upon IR, the phosphorylated gamma H2AX is deposited at sites of DNA breaks. In this assay, 24 h after IR, WT-NPCs display few foci of H2AX, indicating effective DNA repair machinery. On the other hand, A-T-NPCs showed significant gamma H2AX foci at 24 h demonstrating a lack of DNA repair consistent with defective ATM activity. Scale bar, 2 μm indand Scale bar, 20 μm ine. (f) Cells from A-T patients typically display decreased mitochondrial membrane potential. Here, JC-1 staining and quantification showed that both types of A-T-NPCs have significantly decreased mitochondrial membrane potential. Error bars reflect s.e.m. Figure 3: Neural derivatives of A-T hiPSCs display physiological deficits common to A-T cellular phenotype. ( a ) In WT-NPCs, induction of DNA damage by IR (2 Gy) led to phosphorylation of ATM at 30 min, as indicated by immunostaining. Conversely, A-T-NPCs lacked substantial ATM phosphorylation at this time point. Scale bar, 2 μm. ( b ) The phosphorylation of ATM was also measured by FACS. Again, A-T-NPCs failed to induce pATM with this assay as judged by the mean fluorescence intensity across all cells in the culture [29] . ( c ) SMC1, a direct target of ATM phosphorylation, was measured by FACS and presented as mean fluorescence intensity across all cells. A-T-NPCs did not show appreciable levels of SMC1 phosphorylation. ( d , e ) Upon IR, the phosphorylated gamma H2AX is deposited at sites of DNA breaks. In this assay, 24 h after IR, WT-NPCs display few foci of H2AX, indicating effective DNA repair machinery. On the other hand, A-T-NPCs showed significant gamma H2AX foci at 24 h demonstrating a lack of DNA repair consistent with defective ATM activity. Scale bar, 2 μm in d and Scale bar, 20 μm in e . ( f ) Cells from A-T patients typically display decreased mitochondrial membrane potential. Here, JC-1 staining and quantification showed that both types of A-T-NPCs have significantly decreased mitochondrial membrane potential. Error bars reflect s.e.m. Full size image Physiological phenotypes of AT cells in vitro We next sought to determine the physiological consequences of loss of ATM in neural cells including defects in DNA repair and mitochondrial function. Gamma irradiation (IR) is known to cause double-stranded DNA breaks, and these breaks and their subsequent repair can be monitored by the presence of gamma-H2AX, a phosphorylated histone variant involved in DNA repair [30] . WT-NPCs showed very few gamma-H2AX foci-positive cells (?4 foci per nucleus) 24 h after IR, indicating that DNA repair had been successfully completed by that time point [31] ( Fig. 3d ). On the other hand, both lines of A-T-NPCs displayed significant numbers of gamma-H2AX foci-positive cells at this timepoint indicating their failure to properly complete repair of DNA DSBs by 24 h. Similarly, post-mitotic neurons differentiated from WT NPCs showed normal repair kinetics, while neurons differentiated from A-T-NPCs failed in this regard ( Fig. 3e ). Cells from A-T patients have previously been described to have dysfunctional mitochondria by several measures including membrane potential [32] . Using an uptake and release assay with a specialized fluorophore [32] , we found that WT-NPCs display a significantly higher mitochondrial membrane potential than either of the A-T-NPC lines we tested ( Fig. 3f ). In summary, A-T-NPCs and their derived neurons have little detectable ATM activity, do not respond to DNA damage in a timely manner, and have impaired mitochondrial activity, demonstrating that A-T-iPSCs are a useful tool that can recapitulate aspects of A-T pathogenesis in NPCs and terminally differentiated neuronal cells. Rescue of ATM activity in A-T-NPCs with SMRT compounds The two AT-iPSC lines described here represent two distinct types of ATM mutations: A-T-NONS is homozygous for nonsense mutation 103C>T, and A-T-SPL is a compound heterozygote for a splicing mutation 967A>G and a frameshift mutation 3802delG. We have previously described efforts to use compounds that chemically influence translational read-through of premature termination codons (that is, nonsense mutations), to promote production of functional ATM protein in disease cells [11] , [12] , [33] . One molecule previously described to have powerful read-through capacity, despite significant toxicity, is Geneticin (G418). Here, we show that pre-treatment of nonsense mutation A-T-NPCs with G418 partially rescues DNA repair activity 24 hours after IR ( Fig. 4a ). As a negative control, A-T-NPCs lacking a nonsense mutation (A-T-Spl), which would not be expected to respond to G418 treatment, failed to show a reduction of gamma-H2AX foci-positive cells at 24 hours post-IR ( Fig. 4a ). 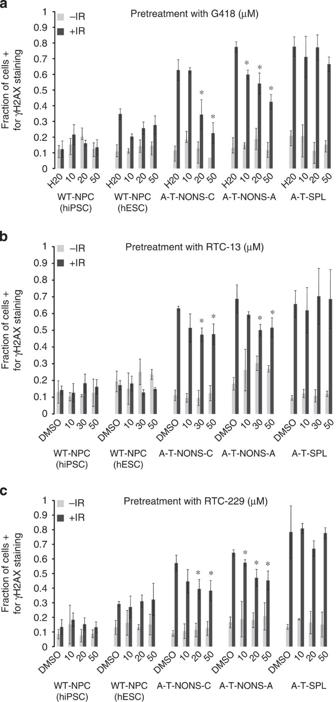Figure 4: SMRT compounds improve DNA repair in A-T-Nons-NPCs. (a) Employing the gamma-H2AX assay (24 h post-IR) in both A-T-Nons sub-lines (C,A) showed improved repair of DSBs following exposure to the RTC, G418. As anticipated, this effect was not observed in WT or A-T-Spl NPCs. (b) Pre-treatment of cells with read-through chemical, RTC-13, similarly resulted in a dose-dependent improvement in DNA repair in both A-T-Nons NPC lines while having no effect on cells lacking nonsense mutations in ATM. (c) When cells were exposed to read-through chemical RTC-229, visualizing gamma-H2AX foci at 24 h post-IR, DNA repair capacity partially improved in both A-T-Nons NPCs but not in the A-T- NPCs with the splicing mutation, a mutation that is not expected to be sensitive to RTCs. At least 200 cells were scored for each condition presented. Error bars represent s.d. across three replicate experiments. Asterisks denote statistically significant withP<0.05 by two-tailed Student’st-test. Figure 4: SMRT compounds improve DNA repair in A-T-Nons-NPCs. ( a ) Employing the gamma-H2AX assay (24 h post-IR) in both A-T-Nons sub-lines (C,A) showed improved repair of DSBs following exposure to the RTC, G418. As anticipated, this effect was not observed in WT or A-T-Spl NPCs. ( b ) Pre-treatment of cells with read-through chemical, RTC-13, similarly resulted in a dose-dependent improvement in DNA repair in both A-T-Nons NPC lines while having no effect on cells lacking nonsense mutations in ATM. ( c ) When cells were exposed to read-through chemical RTC-229, visualizing gamma-H2AX foci at 24 h post-IR, DNA repair capacity partially improved in both A-T-Nons NPCs but not in the A-T- NPCs with the splicing mutation, a mutation that is not expected to be sensitive to RTCs. At least 200 cells were scored for each condition presented. Error bars represent s.d. across three replicate experiments. Asterisks denote statistically significant with P <0.05 by two-tailed Student’s t -test. Full size image As G418 is toxic to cells in culture and in vivo , and is too large to cross the blood–brain barrier, we previously identified alternative SMRT compounds with with a lower toxicity profile [11] . Application of these SMRT compounds to nonsense mutation A-T-NPCs resulted in partial abrogation of the DNA repair defect, although to a somewhat lesser extent than G418 ( Fig. 4b ). However, the lower toxicity profile of the SMRT compounds, when compared with G418, makes them significantly more attractive as potential therapies for genetic disorders arising from nonsense mutations. These data suggest that reprogramming A-T patient cells to a pluripotent state allows a new paradigm for the identification and characterization of SMRT compounds that may prove clinically useful for restoring ATM activity and improving DNA repair capacity. Here we report the generation of iPSCs from A-T patient-derived fibroblasts that carry specific disease causing nonsense mutations, which can be abrogated by SMRT compounds so that their phenotypes at molecular and physiological levels can be assessed. These iPSCs were then used to make neural derivatives (NPCs and neurons) that displayed hallmarks of A-T disease in vitro . We also provide evidence that a γ-H2AX foci assay is a promising way to monitor ATM activity in neural derivatives of A-T-iPSCs before and after exposure to drug candidates (G418, RTC-13 and RTC-229) for treating genetic diseases. Recently, Nayler et al. [34] also reported the generation of A-T-iPSCs with a frameshift deletion, and these cells had a similar cellular phenotype as those described herein. However, the frameshift mutations presented in Nayler et al. [34] preclude correction by current methods. Thus, the neurogenetic model system of A-T that we have developed in this study, when combined with ATM induction by SMRT compounds, provides a unique opportunity to abrogate the A-T neural phenotype and further dissect the pathogenesis of individual mutations. The proof of principle we demonstrate can also be applied to other stem cell models of genetic disease. A-T patient-derived LCLs and Atm knockout mice also have mitochondria dysfunction [32] , [35] , [36] , findings that are consistent with the reduced mitochondrial membrane potential in the A-T-NPCs shown here. In addition, ATM has been shown to be involved in cellular oxidative stress pathways [37] , which are associated with mitochondria via reactive oxygen species. Although ATM protein is localized to this compartment as well, its role in mitochondrial function may or may not be intrinsic to the mitochondrion [38] . Therefore, the data presented here demonstrate that AT-iPSC lines can provide a platform for dissecting the role of ATM in not just DNA repair but also mitochondrial biology, as SMRT compounds restored ATM activity in A-T-NPCs. Loss of PCs is thought to be the major cerebellar defect in A-T patients [16] , [18] . However, the underlying mechanisms remain unclear: is PC loss due to defects in differentiation, migration, apoptosis or interaction with other cell types? The A-T iPSCs described herein are again novel tools for investigating this question as well as the broader question of neural pathogenesis in A-T. This tool also has the advantage of being partially reversible with SMRT compounds to monitor the reversal of ATM deficiency caused by a nonsense mutation. Despite this, the major barrier remains the differentiation from pluripotent stem cells towards PCs, as there is scant evidence that this is possible with current technologies [39] , [40] . This barrier might be inherent to differentiation from human pluripotent stem cells in general, as our previous data have suggested that hPSC differentiation only recapitulates development that occurs in the first trimester of gestation [41] . In the brain, PC migration from the subventricular zone is thought to begin around 16 weeks gestation and continues until after birth [16] , [18] . Therefore, generation of PC from pluripotent stem cells may prove to be difficult until more effective means of modelling the later stages of gestation are developed. Furthermore, culturing cells in two dimensional systems could preclude a bona fide model of A-T in vitro . ‘Ectopic’/‘heterotopic’ PCs have been noted by numerous investigators, consisting mostly of over-migrating PCs in the molecular layer in A-T patients. In addition, PCs have also been noted in the internal granular layer (that is, under-migrating); however, because of the increased cellular density of the internal granular layer, ectopic PCs may be more difficult to discern in this layer [42] . Considering that our cell culture model for NPC specification and differentiation is most similar to time points far earlier than 16 weeks of gestation and that we cannot model PC migration, it is not surprising that the cultured cells in our experiments have not yet yielded any AT-specific changes in neuronal differentiation that would be distinct from comparably differentiated cells derived from WT. Regardless, the data presented here suggest that patient-specific hiPSCs can serve as a valuable tool for the dissection of the molecular pathogenesis of A-T. Generation of A-T iPSC and neural differentiation Two primary fibroblast lines, GM01588 (103C>T) and AG04405 (het. (a)967A>G; (b)3802delG), from patients with A-T were obtained from Coriell Cell Repositories. In all, 1 × 10 5 fibroblasts were plated in a gelatin-coated well of a 6-well plate in MEF media (DMEM/F12+10% FBS). After 8–12 h, the cells were infected with reprogramming lentivirus that harbours polycystronic human Yamanaka factors (Oct4, Klf4, Sox2, cMyc) in DMEM medium containing 10 μg ml −1 of polybrene and incubated overnight at 37 °C in 5% CO 2 incubator. The following day, the viral media was aspirated, replaced with MEF media and cultured for three additional days. Cells were replated on the 5th day onto irradiated MEFs in MEF media. On day 6, the culturing media was changed to human ES media containing DMEM/F12 supplemented with L -glutamine, non-essential amino acids, penicillin–streptomycin, knockout serum replacement (Invitrogen), and 10 ng ml −1 basic FGF. Cells were cultured in hES media until iPSC-like colonies formed. Reprogrammed colonies were further identified by live immunofluorescence staining with TRA1–81 (Chemicon) then mechanically isolated. For early passages, the iPSCs were propagated mechanically, whereas collagenase was used for subsequent passaging. hiPSCs were cultured as described previously in accordance with the UCLA ESCRO [43] , [44] . Neural specification with neural rosette derivation, neuroprogenitor purification and further differentiation to neurons and glia were performed as described previously [41] . Teratoma assay Teratoma Assay was performed by Applied StemCell, Inc. Briefly, hiPSC were sent to Applied StemCell, Inc. A total of 2–4 × 10 6 hiPSCs were injected into kidney capsules and testis of 6-week-old SCID mice. About 8–12 weeks after the injection, teratomas were isolated, fixed in 10% formalin and then embedded in paraffin. Five micron sections were stained with haematoxylin and eosin, and examined for the presence of derivatives of the three germ layers. Karyotyping analysis Karyotyping was performed by Cell Line Genetics as described [44] , [45] . Briefly, Slides were prepared for metaphase analysis according to standard cytogenetic protocols. Cytogenetic analysis was performed on twenty G-banded metaphase cells to assess the presence of chromosomal aberrations. Gene expression-based karyotyping analysis Gene expression-based karyotyping was performed as described [21] , [22] . Affymetrix U133Plus2.0 microarrays were analysed for quality control and outliers removed. For each cell type, probes absent in over 20% of the samples were discarded. In the case of multiple probe sets for any given gene, multiple instances were discarded, so that each gene would be represented by one probeset only. Thus, separate data sets containing a single probeset for each expressed gene were generated for hiPSCs, NPCs and fibroblasts. In order to reduce bias due to low expression levels, values under 50 were collectively raised to this level. In order to further reduce noise in the NPC database, the sum of squares of the relative expression values was calculated for each gene and highly variable genes (SSQ>10) were removed as well. For each sample, the expression value of each gene was divided by the median of the same gene across the entire data set, in order to obtain a comparative value. This median then served as the baseline for examining expression bias. The data were then processed using a freely available CGH analysis software program, CGH-Explorer (heim.ifi.uio.no/bioinf/Projects/CGHExplorer). Gene expression regional bias was detected using the program’s piecewise constant fit algorithm, using a set of parameters as follows: least allowed deviation=0.275–0.3; least allowed aberration size=50–80; winsorize at quantile=0.001; penalty=10–12; threshold=0.01. For each sample in which an aberration was detected, a list of genes that are overexpressed (>1.5-fold, for gains) or under-expressed (<2-fold, for deletions) relative to the median expression of that gene was comprised. In order to test for enrichment of chromosome bands, chromosome arms or full chromosomes, this list was subjected to location enrichment analysis, using the Expander software ( http://acgt.cs.tau.ac.il/expander ). Significance was determined as Bonferroni corrected P -values lower than 1.0E-4, which is the default value of the Expander program. Immunostaining and western blot Cells on coverslips were washed with PBS, fixed in 4% paraformaldehyde for 15 min at room temperature, blocked for 1 h at room temperature with 10% serum and 0.1% Triton-X-100, then incubated overnight at 4 °C with primary antibodies. Following primary antibody incubation, the coverslips were incubated with Alexa Fluor secondary antibodies (Invitrogen) at room temperature for 1 h and mounted in Prolong Gold with DAPI (Invitrogen). Imaging was performed on Zeiss Axio Imager A1 or Zeiss LSM780 confocal microscope. Antibodies used included: mouse anti-OCT3/4 (1:100, Santa Cruz Biotechnology Inc.), rabbit anti-SOX2 (1:300, Cell Signaling Technology), rabbit anti-Nanog (1:100, Cell Signaling Technology), mouse anti-Tra-1–81 (1:250, Chemicon), mouse anti-NESTIN (1:1,000, Neuromics), mouse anti-MAP2 (1:500, Abcam), chicken anti-GFAP (1:2,000 Abcam), rabbit anti-ATM (1:200 for Immunofluorescence; 1:5,000 for western blot, Abcam). Western blot analysis was performed using standard procedures as described [46] . Gene expression profiling Gene expression profiling was performed on Affymetrix Human HG-U133 2.0 Plus microarrays as described previously [41] . CEL files were imported into genespring and normalized to the mean of all samples with the robust multichip algorithm (RMA). Probe sets that were not expressed at a raw value of >50 in at least 10% of samples were eliminated from further analysis. Hierarchical clustering was performed by and samples were linked by complete linkage with complete Euclidian clustering analysis. DNA damage and repair assay The gamma-H2AX and ATM-pS1981 foci staining have been previously described [29] , [31] , [47] . Briefly, cells on coverslips were irradiated with 2 Gy using a Mark IV Cs-137 gamma irradiation source (dose rate ~4.5 Gy min −1 ). After irradiation, cells were returned to the incubator for 30 min (ATMpS1981) or for 24 h (gamma-H2AX) before being fixed with 4% paraformaldehyde. Cells were permeabilized with 0.5% Triton-X-100 in PBS. Cells were incubated with primary antibodies followed by fluorescent secondary antibodies after first blocking with 10% FBS. Once the cells were stained with the appropriate antibodies, coverslips were transferred to microscope slides and mounted with Prolong Gold mounting medium with DAPI (Life Technologies). Coverslips were sealed and later imaged using an Olympus fluorescent microscope equipped with an AxioVision camera and acquisition software. The antibodies used were: gamma-H2AX (mouse, 1:300, Millipore), ATM-pS1981 (mouse, 1:300, Cell Signaling), SOX2 (rabbit, 1:400, Cell Signaling), Alexa-fluor488 (anti-mouse, 1:400, Invitrogen) and Alexa-fluor568 (anti-rabbit, 1:500, Invitrogen). At least 200 nuclei were evaluated for each sample and nuclei were scored as positive (?4 foci per nucleus) or negative (<4 foci per nucleus). The results are reported as fraction of cells positive for ?4 loci of gamma-H2AX staining. Statistical significance was determined using two-tailed Student’s t -test and P <0.05 was considered significant (indicated by *). FACS analysis of ATM activity ATM activity was monitored by phosphorylation of ATM at S1981 (1:100, Cell Signaling) and SMC1 at S966 (1:100, Novus Biologics) as previously described [29] . Briefly, cells were irradiated with 10 Gy using a Mark IV Cs-137 gamma-irradiation source (dose rate ~4.5 Gy min −1 ) followed by collection and fixation 30 min after irradiation. A double-fixation method using the Invitrogen fix and perm kit and cold methanol was performed according to manufacturers’ protocol. Cells were then stained with primary antibodies for 1 h at room temperature and FITC secondary antibody (Jackson Immunologics) at 1:100 for 45 min at room temperature. Staining intensities (FL-1) were then acquired by FACS (Beckson Dickerson) and analysed using FlowJo (TreeStar Inc.). Measurement of mitochondrial membrane potential JC-1 (5,5′,6,6′-tetrachloro-1,1′,3,3′-tetraethylbenzimidazolylcarbocyanine iodide) (Molecular Probes) is a non-toxic fluorescence probe and can be taken up by cells and specifically accumulated inside the mitochondria because of its cationic and lipophilic nature in proportion to the magnitude of membrane potential (ΔΨm). When JC-1 exists as a monomer, it fluoresces green and in healthy mitochondria, it forms aggregates which fluoresce red. Therefore, the ratio of ’red‘ to ’green‘ fluorescence is used to detect ΔΨm changes. Cells were collected in warm media at approximately 1 × 10 6 cells per ml and stained with 2 μM JC-1 under normal growth conditions for 30 min. As a positive control, cells were treated with 50 μM of the membrane potential disrupter CCCP (carbonyl cyanide 3-chlorophenylhydrazone, supplied with the kit) for 5 min before JC-1 staining. The drug treatment was used to show that JC-1 response was membrane potential sensitive. After staining, cells were pelleted by centrifugation and resuspended in 500 μl of PBS and immediately analysed using BD FACS Calibur flow cytometer. Red and green fluorescent measurements where obtained using 488 nm excitation, with emissions of 530 nm for green and 585 nm for red. SMRT compound treatment Cells were treated as previously described [11] , at concentrations indicated in the figures. Other samples were mock treated with the vehicle. Water is the vehicle for G418 (Mediatech), while DMSO was used for RTC-13 and RTC-229. Stock solutions were diluted in culture media to the reported concentration and added to cells on coverslips in 24-well plates. This constituted day 0 of treatment and this process was repeated on day 2 to feed the cells with fresh media containing read-through compounds. Cells were irradiated for the gamma-H2AX assay on day 4 as described above. Accession Code: Sequences for the microarray data in Supplementary Data 1 have been deposited in the Gene Expression Omnibus database under the accession number GSE45030 . How to cite this article: Lee, P. et al. SMRT compounds abrogate cellular phenotypes of ataxia telangiectasia in neural derivatives of patient-specific hiPSCs. Nat. Commun. 4:1824 doi: 10.1038/ncomms2824 (2013).